FOXL2 posttranslational modifications mediated by GSK3β determine the growth of granulosa cell tumours Approximately 97% of patients with ovarian granulosa cell tumours (GCTs) bear the C134W mutation in FOXL2; however, the pathophysiological mechanism of this mutation is unknown. Here we report how this mutation affects GCT development. Sequential posttranslational modifications of the C134W mutant occur where hyperphosphorylation at serine 33 (S33) by GSK3β induces MDM2-mediated ubiquitination and proteasomal degradation. In contrast, S33 of wild-type FOXL2 is underphosphorylated, leading to its SUMOylation and stabilization. This prominent hyperphosphorylation is also observed at S33 of FOXL2 in GCT patients bearing the C134W mutation. In xenograft mice, the S33 phosphorylation status correlates with the oncogenicity of FOXL2, and the inhibition of GSK3β efficiently represses GCT growth. These findings reveal a previously unidentified regulatory mechanism that determines the oncogenic attributes of the C134W mutation via differential posttranslational modifications of FOXL2 in GCT development. Ovarian granulosa cell tumours (GCTs) are a distinct subset of malignant ovarian cancers that originate from the sex cord-stromal cells, and the adult type accounts for the majority of GCTs [1] . The prominent characteristics of GCTs are a slow and indolent disease progression and a propensity for frequent, long delays to recurrence [1] , [2] . The molecular pathogenesis of adult-type GCTs has been largely unknown until a recent discovery of a missense point mutation, c.402C→G (p.C134W) in the FOXL2 gene [3] . The C134W mutation was exclusively detected in 97% of adult-type GCTs in a whole-transcriptome paired-end RNA sequencing study [3] . Efforts have been made to address the role of the C134W mutation in GCT by investigating its effects on target gene regulation [4] , [5] , [6] , [7] . We previously determined that compared with the wild-type (WT) FOXL2 protein, the C134W mutant is less efficient in conveying the apoptosis signalling associated with its compromised transcriptional activities to death receptors, including TNF-R1 (tumour necrosis factor-receptor 1) and FAS (CD95/APO-1) [8] . However, the underlying molecular mechanism of the C134W mutation in GCT development is not known. The evolutionarily conserved forkhead (FH) domain-containing transcription factor FOXL2 is highly expressed in ovarian granulosa cells [9] . Familial mutations in FOXL2 cause blepharophimosis-ptosis-epicanthus inversus syndrome (OMIM 110100), characterized by malformations of the eyelid and/or premature ovarian failure [10] . FoxL2 lacZ homozygous mutant female mice are infertile owing to ovarian failure resulting from the lack of granulosa cell differentiation [11] , [12] . Moreover, FOXL2 ablation reprogrammes adult ovarian follicles into testicular cells, suggesting that FOXL2 is required to prevent the transdifferentiation of the ovary to the testis [13] . These observations suggest that elucidating the pathophysiology of GCT development through the C134W mutation could allow for an understanding of both the fundamentals of FOXL2 in maintaining normal ovarian physiology and the molecular mechanisms of GCT development. Posttranslational modifications (PTMs) of FOXL2 have been reported, indicating the presence of phosphorylated FOXL2 peptides [14] , FOXL2 phosphorylation by LATS1 (ref. 15 ), and enhanced FOXL2 stability and transcriptional activity on SUMOylation [14] , [16] , [17] . However, at present, very little is known regarding the mechanism and functional importance of crosstalk between FOXL2 PTMs that fine tune the outcomes of signalling pathways in ovarian physiology. For these reasons, we investigated the physiological role of FOXL2 PTMs using the C134W mutation as a pathological model. On the basis of our finding of differential phosphorylation of serine 33 (S33) on WT FOXL2 and the C134W mutant using tandem mass spectrometry, we investigate the physiological roles of PTMs of FOXL2. In this study, we discovered a cascade of FOXL2 PTMs in which S33 is phosphorylated by glycogen synthase kinase-3β (GSK3β), allowing for MDM2-mediated FOXL2 ubiquitination and proteasomal degradation. We observed this prominent S33 phosphorylation in GCT patients harbouring the C134W mutation and further validated the hyperphosphorylation and oncogenicity by the C134W mutation in a xenograft mouse model. Together, our findings suggest that differential PTMs between WT and C134W FOXL2 contribute to the growth of GCTs. The identification of FOXL2 phosphorylation by GSK3β at S33 We performed mass spectrometry analysis of the immunoprecipitated WT and C134W FOXL2 proteins overexpressed in 293T cells ( Supplementary Fig. S1a ). This analysis and that of the FOXL2 proteome, which was performed via liquid chromatography/mass spectrometry ( Supplementary Fig. S1b ), allowed us to identify two phosphorylation sites (23TVKEPEGPPPpS33PGK36 and 216ASCQMAAAAAAAAAAAAAAGPGpS238PGAAAVVK246; Supplementary Tables S1 and S2 ; Supplementary Fig. S2a,b ). The comparative sequence analysis of FOXL2 homologues in other species was performed to find the potential modification sites, S33 and a set of lysine (K) residues at 25, 36, 48 and 54, conserved in all of the mammals examined ( Fig. 1a ). An in silico prediction of kinases (GPS2.1; http://gps.biocuckoo.org ) suggested that S33 is a potential substrate of CDK1, GSK3β, ERK, mitogen-activated protein kinase and c-Jun amino-terminal kinase( Supplementary Fig. 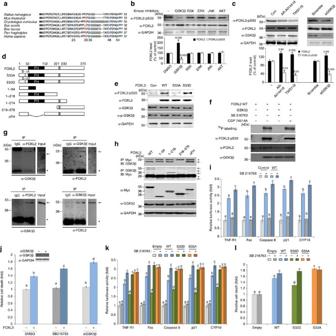Figure 1: GSK3β interacts with FOXL2 and phosphorylates its serine 33 residue, leading to the modulation of FOXL2 function. (a) The alignment of mammalian FOXL2 proteins, encompassing S33 (red) and the proximal lysine (K; blue) residues of FOXL2 is shown. (b) Changes of S33 phosphorylation by kinase inhibitors were determined using the phospho-S33-specific FOXL2 antibody. After the KGN cells were transfected with Myc-FOXL2, they were incubated with 10 μM of the GSK3β (SB 216763), RSK (SL0101), ERK (U0126), JNK (SP600125) or AKT (LY 294002) inhibitors, or 0.1% dimethyl sulphoxide (DMSO) as a solvent control for 18 h. Quantitative analyses of the S33-phosphorylated FOXL2 and FOXL2 levels are shown (n=5; lower panel). (c) KGN cells were transfected with Myc-FOXL2 and incubated with 10 μM AR-A014418 or TWS119 (left panel), or transfected with scramble or GSK3β siRNA (200 nM; right panel) for 18 h. Quantitative analyses of S33-phosphorylated FOXL2 and FOXL2 levels are shown (n=3; lower panel). (d) The FOXL2 mutants were generated as indicated. (e) Immunoblot analyses of S33A and S33D FOXL2 mutants are shown. (f)In vitrokinase assay was performed. Purified FOXL2 protein (2 μg) was incubated with active GSK3β (0.05 μg) with or without 10 μM GSK3β inhibitor (SB 216763) or CDK1 inhibitor (CGP 74514A). (g) The endogenous interaction (upper panels) between FOXL2 and GSK3β, and thein vitrointeraction (lower panels) of recombinant FOXL2 (2 μg) and active GSK3β (0.1 μg) were analysed following immunoprecipitation. The arrows indicate expected proteins, whereas asterisks represent nonspecific bands throughout the figures. (h) Truncated Myc-tagged FOXL2 mutants were transfected into KGN cells, and their binding capacities were assessed using immunoprecipitation. (i,k) KGN cells were transfected with an empty vector, FOXL2 WT, S33A or S33D with indicated promoters in the presence of 10 μM SB 216763 or 0.1% DMSO. (j,l) KGN cells were transfected with FOXL2s or transfected with scramble or GSK3β siRNA for 18 h. All of the results (means±s.e.m.) are from at least three independent experiments performed in triplicate. The statistically significant values are indicated with asterisks or different letters (P<0.05; Student’st-test forbandcor Student–Newman–Keuls test fori–l). S3a ), whereas Calmodulin 1 was also identified in the mass spectrometry analysis of the immunoprecipitated WT FOXL2 ( Supplementary Table S1 ) Figure 1: GSK3β interacts with FOXL2 and phosphorylates its serine 33 residue, leading to the modulation of FOXL2 function. ( a ) The alignment of mammalian FOXL2 proteins, encompassing S33 (red) and the proximal lysine (K; blue) residues of FOXL2 is shown. ( b ) Changes of S33 phosphorylation by kinase inhibitors were determined using the phospho-S33-specific FOXL2 antibody. After the KGN cells were transfected with Myc-FOXL2, they were incubated with 10 μM of the GSK3β (SB 216763), RSK (SL0101), ERK (U0126), JNK (SP600125) or AKT (LY 294002) inhibitors, or 0.1% dimethyl sulphoxide (DMSO) as a solvent control for 18 h. Quantitative analyses of the S33-phosphorylated FOXL2 and FOXL2 levels are shown ( n =5; lower panel). ( c ) KGN cells were transfected with Myc-FOXL2 and incubated with 10 μM AR-A014418 or TWS119 (left panel), or transfected with scramble or GSK3β siRNA (200 nM; right panel) for 18 h. Quantitative analyses of S33-phosphorylated FOXL2 and FOXL2 levels are shown ( n =3; lower panel). ( d ) The FOXL2 mutants were generated as indicated. ( e ) Immunoblot analyses of S33A and S33D FOXL2 mutants are shown. ( f ) In vitro kinase assay was performed. Purified FOXL2 protein (2 μg) was incubated with active GSK3β (0.05 μg) with or without 10 μM GSK3β inhibitor (SB 216763) or CDK1 inhibitor (CGP 74514A). ( g ) The endogenous interaction (upper panels) between FOXL2 and GSK3β, and the in vitro interaction (lower panels) of recombinant FOXL2 (2 μg) and active GSK3β (0.1 μg) were analysed following immunoprecipitation. The arrows indicate expected proteins, whereas asterisks represent nonspecific bands throughout the figures. ( h ) Truncated Myc-tagged FOXL2 mutants were transfected into KGN cells, and their binding capacities were assessed using immunoprecipitation. ( i , k ) KGN cells were transfected with an empty vector, FOXL2 WT, S33A or S33D with indicated promoters in the presence of 10 μM SB 216763 or 0.1% DMSO. ( j , l ) KGN cells were transfected with FOXL2s or transfected with scramble or GSK3β siRNA for 18 h. All of the results (means±s.e.m.) are from at least three independent experiments performed in triplicate. The statistically significant values are indicated with asterisks or different letters ( P <0.05; Student’s t -test for b and c or Student–Newman–Keuls test for i – l ). Full size image We generated a polyclonal antibody that recognizes the phospho-S33 residue, which was designated as FOXL2-pS33 antibody. With this antibody, we determined that the phosphorylation of S33 was specifically diminished in the presence of the GSK3β inhibitor SB 216763, with a concomitant increase in FOXL2 levels ( Fig. 1b and Supplementary Fig. S3b ). Other GSK3β inhibitors (AR-A014418 and TWS119) and small interfering RNA (siRNA) treatment against GSK3β in KGN cells also attenuated S33 phosphorylation ( Fig. 1c ). To delineate the mechanisms that underlie this phosphorylation, various FOXL2 mutants were produced ( Fig. 1d ). The S33A mutant was negative for S33 phosphorylation, whereas the S33D mutant behaved as S33-hyperphosphorylated FOXL2 ( Fig. 1e ). We found that the FOXL2-pS33 antibody recognizes the S33D mutant in a phosphorylation-dependent manner ( Supplementary Fig. S3c ). An in vitro kinase assay using purified recombinant proteins revealed that GSK3β indeed phosphorylated FOXL2 at S33 ( Fig. 1f ). In addition, the S33 phosphorylation of FOXL2 was markedly reduced below the detection limit in the presence of the GSK3β inhibitor SB 216763 but not by the CDK1 inhibitor CGP 74514A ( Fig. 1f ). Moreover, FOXL2 physically interacted with active GSK3β, as was indicated by immunoprecipitation ( Fig. 1g ), whereas the inactive form of GSK3β (phosphorylated S9) did not interact with FOXL2 ( Supplementary Fig. S3d ). Immunoprecipitation assays with various FOXL2 mutants as shown in Fig. 1d indicated that GSK3β bound to the N-terminal region between amino acids (aa) 1–52, within the FOXL2 sequence that encompasses S33 ( Fig. 1h ). The stoichiometry of GSK3β-mediated FOXL2 phosphorylation was ~0.1 mol of 32 P incorporated/mol of FOXL2 when measured using purified proteins ( Supplementary Fig. S3e ). Diminished FOXL2 activities by S33 phosphorylation FOXL2 overexpression transactivated target genes including TNF-R1 , Fas , Caspase 8 , p21 and CYP19 ( aromatase ) promoters [4] , [8] , [18] , [19] , and transcriptional activation of these genes was further increased in the presence of SB 216763 ( Fig. 1i ). The cell death activity of FOXL2 was also enhanced in KGN cells that were incubated with either SB 216763 or GSK3β-specific siRNA ( Fig. 1j ). When GSK3β activity is uninhibited, the phosphorylation-resistant mutant (S33A) increased transcriptional and apoptotic activities compared with the WT FOXL2 protein, whereas the S33D mutant exhibited reduced activities relative to the levels that were observed with the WT protein ( Fig. 1k,l ). Addition of SB 216763 significantly increased the activation of target genes and cell death activity in cells that expressed the S33D mutant compared with the compound’s negligible effect on the S33A mutant ( Fig. 1k,l ). The S33D mutant also responded to GSK3β inhibition, implying the ability of GSK3β to phosphorylate the S33D mutant. We found that phosphorylation of the S33D mutant is inhibited by SB 216763 ( Supplementary Fig. S3f ). These results indicate that the functional activities of FOXL2 decrease following GSK3β-mediated S33 phosphorylation. S33 phosphorylation alters the degradation of FOXL2 To investigate how GSK3β-mediated S33 phosphorylation reduces FOXL2 activities, we compared protein stability with respect to the status of S33 phosphorylation. As shown in Fig. 2a , the stability of FOXL2 was enhanced in the presence of the GSK3β inhibitor. Furthermore, we observed that FOXL2 was ubiquitinated and degraded by the proteasome and that its ubiquitination was inhibited by SB 216763 ( Fig. 2b ). Compared with WT FOXL2, the S33A mutant exhibited enhanced overall protein stability, whereas the stability of S33D FOXL2 was reduced ( Fig. 2c ). Moreover, reduced or augmented ubiquitination was observed for the S33A or S33D mutants, respectively, in comparison with WT ( Fig. 2d ). These variable stabilities of FOXL2 proteins leading to their different expression levels mainly contributed to differential transcriptional activation of target genes of FOXL2 as shown in Supplementary Fig. S3g . Interestingly, the opposite pattern was observed for FOXL2 SUMOylation, that is, there was an enhancement or reduction in FOXL2 SUMOylation when the S33A or S33D mutants were overexpressed, respectively ( Fig. 2d ). FOXL2 specifically bound to SUMO1 but not to SUMO2 or SUMO3 ( Supplementary Fig. S3h ). The E2 SUMO-conjugating enzyme UBC9, which is a known FOXL2-interacting protein that enhances FOXL2 SUMOylation [16] , interacted more weakly with the S33D mutant protein but more strongly with S33A compared with the WT protein; this effect was followed by changes in the SUMOylation of these mutant proteins ( Fig. 2e ). Moreover, UBC9 overexpression significantly attenuated the ubiquitination of WT but not of mutant proteins ( Fig. 2e ). Thus, these data imply that S33 acts as a phosphodegron that stimulates FOXL2 ubiquitination and degradation but hinders its SUMOylation. 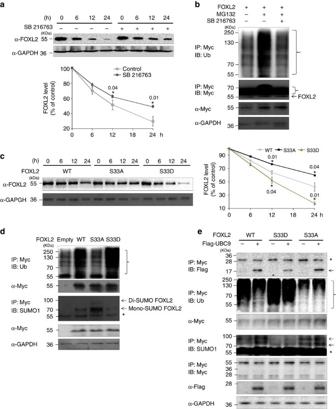Figure 2: GSK3β-induced FOXL2 S33 phosphorylation affects FOXL2 ubiquitination and SUMOylation. (a) KGN cells were transfected with FOXL2, incubated with 10 μM SB 216763 or 0.1% dimethyl sulphoxide in the presence of cycloheximide (10 μg ml−1) and collected at the indicated time points. Western blot analyses were then performed (n=3). The data (means±s.e.m.) are normalized to glyceraldehydes 3-phosphate dehydrogenase (GAPDH) expression, and the FOXL2 expression levels are presented as percentages of the control. The statistically significant values are indicated with asterisks (P<0.05; Student’st-test). (b) Myc-FOXL2-transfected KGN cells were incubated with 50 μM MG132 and 10 μM SB 216763, and then immunoprecipitated with anti-Myc. Western blot analysis was then performed using an anti-ubiquitin antibody. The brace indicates ubiquitinated FOXL2. (c) The effect of S33 phosphorylation on FOXL2 stability was assessed as described ina. (d) Myc-tagged FOXL2 WT, S33A or S33D-coding plasmids were co-transfected with the HA-SUMO1 plasmid in the presence of MG132 (50 μM). The lysates were immunoprecipitated with anti-Myc antibody and western blot analysis was subsequently performed. (e) The differential interaction of UBC9 with WT, S33D or S33A FOXL2, and the effects of UBC9 on ubiquitination and SUMOylation of these proteins were assessed. Each FOXL2 protein was overexpressed with or without Flag-tagged UBC9 in the presence of 50 μM of MG132 and immunoprecipitates were immunoblotted. Figure 2: GSK3β-induced FOXL2 S33 phosphorylation affects FOXL2 ubiquitination and SUMOylation. ( a ) KGN cells were transfected with FOXL2, incubated with 10 μM SB 216763 or 0.1% dimethyl sulphoxide in the presence of cycloheximide (10 μg ml −1 ) and collected at the indicated time points. Western blot analyses were then performed ( n =3). The data (means±s.e.m.) are normalized to glyceraldehydes 3-phosphate dehydrogenase (GAPDH) expression, and the FOXL2 expression levels are presented as percentages of the control. The statistically significant values are indicated with asterisks ( P <0.05; Student’s t -test). ( b ) Myc-FOXL2-transfected KGN cells were incubated with 50 μM MG132 and 10 μM SB 216763, and then immunoprecipitated with anti-Myc. Western blot analysis was then performed using an anti-ubiquitin antibody. The brace indicates ubiquitinated FOXL2. ( c ) The effect of S33 phosphorylation on FOXL2 stability was assessed as described in a . ( d ) Myc-tagged FOXL2 WT, S33A or S33D-coding plasmids were co-transfected with the HA-SUMO1 plasmid in the presence of MG132 (50 μM). The lysates were immunoprecipitated with anti-Myc antibody and western blot analysis was subsequently performed. ( e ) The differential interaction of UBC9 with WT, S33D or S33A FOXL2, and the effects of UBC9 on ubiquitination and SUMOylation of these proteins were assessed. Each FOXL2 protein was overexpressed with or without Flag-tagged UBC9 in the presence of 50 μM of MG132 and immunoprecipitates were immunoblotted. Full size image MDM2 is the E3 ubiquitin ligase for lysine 25 of FOXL2 To identify the E3 ubiquitin ligase that ubiquitinates FOXL2, we examined the interaction of different E3 ligases with FOXL2. As shown in Fig. 3a , FOXL2 associated with endogenous MDM2 protein but not with other ligases, including ARFBP1, SKP2 and β-TrCP. Forced MDM2 expression significantly decreased FOXL2, whereas other E3 ligases did not alter the FOXL2 level ( Fig. 3b ). Ectopic MDM2 expression enhanced FOXL2 ubiquitination in combination with a concomitant decrease in the FOXL2 level, whereas either overexpression of MDM2 mutant lacking its acidic domain critical for ligase activity (Δ209–274) [20] or knockdown of MDM2 prevented the effective ubiquitination of FOXL2 ( Fig. 3c ). Moreover, the MDM2 inhibitor trans-4-iodo-4′-boranyl-chalcone efficiently blocked the increase in FOXL2 ubiquitination that was elicited by MDM2 overexpression ( Fig. 3d ). Endogenous FOXL2 and MDM2 proteins physically associated in KGN cells ( Fig. 3e ). Analysis of cells that expressed truncated FOXL2 mutants indicated that this association was likely to be mediated by the sequence between aa 54 and 94, within the FH domain ( Fig. 3f ). The FOXL2 S33D mutant exhibited a stronger interaction with MDM2, whereas the S33A mutant showed a weaker interaction ( Fig. 3g ). Similarly, MDM2 overexpression clearly decreased the expression level of S33D, whereas the level of S33A was unaffected ( Fig. 3h ). In vitro ubiquitination and SUMOylation assays confirmed that GSK3β-mediated S33 phosphorylation stimulated FOXL2 ubiquitin conjugation but attenuated FOXL2 SUMOylation ( Fig. 3i ). To identify the residues involved in the S33 phosphorylation-sensitive ubiquitin and SUMO conjugations, each lysine residue of FOXL2 proximal to S33 was mutated to arginine (R), and changes in the expression of each mutant following forced MDM2 expression were analysed. The MDM2-induced degradation of FOXL2 protein was significantly blocked in the K25R mutant compared with other mutants ( Fig. 3j ), suggesting that K25 is a plausible acceptor site for ubiquitin. 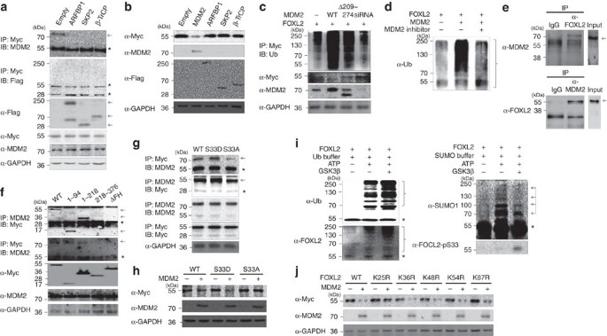Figure 3: MDM2 is the FOXL2 E3 ligase that preferentially interacts with S33-phosphorylated FOXL2 and enhances FOXL2 ubiquitination. (a) Following the transfection of KGN cells with the indicated plasmids, the interaction of MDM2 with FOXL2 was confirmed using immunoprecipitation and western blot analysis. (b) MDM2 as the E3 ligase that is responsible for FOXL2 degradation was identified. KGN cells were transfected with the indicated plasmids, and the change in FOXL2 expression level was assessed using immunoblot analysis. (c) The modulation of FOXL2 ubiquitination by MDM2 was evaluated. Overexpression of WT MDM2 or MDM2 mutant lacking its acidic domain critical for ligase activity (Δ209–274) or knockdown of MDM2 were performed. Myc-tagged FOXL2 was immunoprecipitated with anti-Myc antibody, and immunoprecipitates were immunoblotted with anti-Ubiquitin antibody. (d) MDM2-mediated FOXL2 ubiquitination was confirmedin vitro. Recombinant FOXL2 was incubated with a reaction buffer that contained MDM2 (0.3 μg) or 10 nM trans-4-iodo-4′-boranyl-chalcone. (e) The endogenous interaction of MDM2 with FOXL2 proteins was determined using immunoprecipitation. (f) The MDM2-binding region of FOXL2 was assessed using immunoprecipitation following the overexpression of truncated FOXL2-coding plasmids. (g) The effect of S33 phosphorylation on binding of MDM2 to FOXL2 was assessed using immunoprecipitation. (h) The effect of S33 phosphorylation on MDM2-mediated FOXL2 stability was determined using immunoblotting. (i) Recombinant FOXL2 (2 μg) and active GSK3β (0.05 μg) were incubated with either ubiquitinylation buffer (upper panel) or SUMOylation buffer (lower panel) in the presence or absence of ATP. The arrows indicate SUMOylated FOXL2s. (j) The lysine (K) residue(s) of FOXL2 that were involved in MDM2-mediated ubiquitination were determined after the KGN cells were transfected with mutated FOXL2 and MDM2. Asterisk indicates nonspecific bands. Figure 3: MDM2 is the FOXL2 E3 ligase that preferentially interacts with S33-phosphorylated FOXL2 and enhances FOXL2 ubiquitination. ( a ) Following the transfection of KGN cells with the indicated plasmids, the interaction of MDM2 with FOXL2 was confirmed using immunoprecipitation and western blot analysis. ( b ) MDM2 as the E3 ligase that is responsible for FOXL2 degradation was identified. KGN cells were transfected with the indicated plasmids, and the change in FOXL2 expression level was assessed using immunoblot analysis. ( c ) The modulation of FOXL2 ubiquitination by MDM2 was evaluated. Overexpression of WT MDM2 or MDM2 mutant lacking its acidic domain critical for ligase activity (Δ209–274) or knockdown of MDM2 were performed. Myc-tagged FOXL2 was immunoprecipitated with anti-Myc antibody, and immunoprecipitates were immunoblotted with anti-Ubiquitin antibody. ( d ) MDM2-mediated FOXL2 ubiquitination was confirmed in vitro . Recombinant FOXL2 was incubated with a reaction buffer that contained MDM2 (0.3 μg) or 10 nM trans-4-iodo-4′-boranyl-chalcone. ( e ) The endogenous interaction of MDM2 with FOXL2 proteins was determined using immunoprecipitation. ( f ) The MDM2-binding region of FOXL2 was assessed using immunoprecipitation following the overexpression of truncated FOXL2-coding plasmids. ( g ) The effect of S33 phosphorylation on binding of MDM2 to FOXL2 was assessed using immunoprecipitation. ( h ) The effect of S33 phosphorylation on MDM2-mediated FOXL2 stability was determined using immunoblotting. ( i ) Recombinant FOXL2 (2 μg) and active GSK3β (0.05 μg) were incubated with either ubiquitinylation buffer (upper panel) or SUMOylation buffer (lower panel) in the presence or absence of ATP. The arrows indicate SUMOylated FOXL2s. ( j ) The lysine (K) residue(s) of FOXL2 that were involved in MDM2-mediated ubiquitination were determined after the KGN cells were transfected with mutated FOXL2 and MDM2. Asterisk indicates nonspecific bands. Full size image Regulation of FOXL2 stability via ubiquitin and SUMO Given that the phosphorylation status of S33 differentially affects FOXL2 ubiquitination and SUMOylation ( Fig. 2d ), we next sought to elucidate the reciprocal regulatory mechanism in the PTMs of FOXL2. WT FOXL2 ubiquitination was increased on ubiquitin overexpression and FOXL2 SUMOylation was increased following SUMO1 overexpression ( Fig. 4a ; lanes 1 versus 2 and 1 versus 3). Intriguingly, FOXL2 ubiquitination was significantly decreased in the presence of SUMO1, whereas SUMO conjugation of FOXL2 was not further affected by ubiquitin ( Fig. 4a ; lanes 2 versus 4 and 3 versus 4), suggesting that SUMOylated FOXL2 is resistant to ubiquitin conjugation. Compared with WT FOXL2, the S33A mutant was less ubiquitinated and its ubiquitination level was reduced by SUMO1 expression ( Fig. 4a ; lanes 1 versus 5 and 6 versus 8). In contrast, the S33D mutant was heavily ubiquitinated and its ubiquitin conjugation was not significantly affected by SUMO1 ( Fig. 4a ; lanes 1 versus 9 and 10 versus 12). In addition, MDM2-induced FOXL2 ubiquitination was attenuated on UBC9 overexpression ( Fig. 4b ; lane 2 versus 4). However, UBC9-induced FOXL2 SUMOylation was unaffected by MDM2 ( Fig. 4b ; lane 3 versus 4). Taken together, these results indicate that the SUMOylation of FOXL2 inhibits FOXL2 ubiquitination, whereas forced ubiquitination is unable to affect SUMOylation, implying a hierarchical regulation between ubiquitination and SUMOylation. 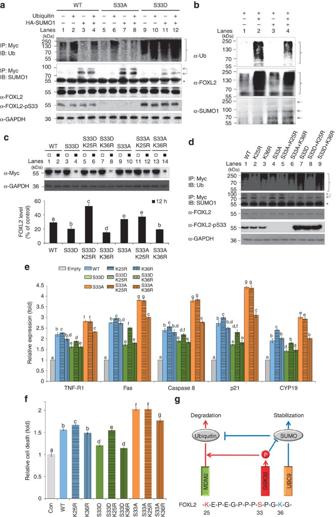Figure 4: The contrasting effects of S33 phosphorylation-dependent regulation of FOXL2 ubiquitination and SUMOylation. (a) Myc-tagged WT FOXL2, S33A or S33D were overexpressed in KGN cells with ubiquitin, SUMO1 or both in the presence of MG132 (50 μM). The lysates were immunoprecipitated and western blot analyses were performed using the respective antibodies. (b) The effect of FOXL2 SUMOylation on its ubiquitination was confirmedin vitroas described in the legend ofFig. 3i. Recombinant FOXL2 (2 μg) was incubated with MDM2 (0.3 μg), UBC9 (0.5 μg) or both for 30 min, and the changes in FOXL2 ubiquitination and SUMOylation were determined using western blotting. (c) Changes in protein stability on introduction of mutations in FOXL2 were determined by immunoblotting following overexpression of each protein for 12 h in the presence of cycloheximide (50 μM). (d) Changes in ubiquitination and SUMOylation were assessed following overexpression of each FOXL2 mutant in the presence of 50 μM MG132. (e) Changes in the transcriptional activities of FOXL2 mutants were assessed using real-time PCR with a cDNA library that was synthesized from RNA that was isolated from KGN cells separately overexpressing each mutant protein. Results (means±s.e.m.) are from three independent experiments performed in triplicate. The statistically significant values are indicated with different letters (P<0.05; Student–Newman–Keuls test). (f) The effects on cell death activity of the FOXL2 mutants were determined and analysed following the overexpression of each mutant according toe. (g) A proposed model is shown in which GSK3β-mediated FOXL2 S33 phosphorylation defines the path to its subsequent PTM modifications, namely ubiquitination or SUMOylation. Asterisk indicates nonspecific bands. Figure 4: The contrasting effects of S33 phosphorylation-dependent regulation of FOXL2 ubiquitination and SUMOylation. ( a ) Myc-tagged WT FOXL2, S33A or S33D were overexpressed in KGN cells with ubiquitin, SUMO1 or both in the presence of MG132 (50 μM). The lysates were immunoprecipitated and western blot analyses were performed using the respective antibodies. ( b ) The effect of FOXL2 SUMOylation on its ubiquitination was confirmed in vitro as described in the legend of Fig. 3i . Recombinant FOXL2 (2 μg) was incubated with MDM2 (0.3 μg), UBC9 (0.5 μg) or both for 30 min, and the changes in FOXL2 ubiquitination and SUMOylation were determined using western blotting. ( c ) Changes in protein stability on introduction of mutations in FOXL2 were determined by immunoblotting following overexpression of each protein for 12 h in the presence of cycloheximide (50 μM). ( d ) Changes in ubiquitination and SUMOylation were assessed following overexpression of each FOXL2 mutant in the presence of 50 μM MG132. ( e ) Changes in the transcriptional activities of FOXL2 mutants were assessed using real-time PCR with a cDNA library that was synthesized from RNA that was isolated from KGN cells separately overexpressing each mutant protein. Results (means±s.e.m.) are from three independent experiments performed in triplicate. The statistically significant values are indicated with different letters ( P <0.05; Student–Newman–Keuls test). ( f ) The effects on cell death activity of the FOXL2 mutants were determined and analysed following the overexpression of each mutant according to e . ( g ) A proposed model is shown in which GSK3β-mediated FOXL2 S33 phosphorylation defines the path to its subsequent PTM modifications, namely ubiquitination or SUMOylation. Asterisk indicates nonspecific bands. Full size image To further address the relationship between the three different PTMs of FOXL2, additional site-directed double mutants that contained substitutions at both S33 and K25 or K36 were generated. The decreased stability of S33D FOXL2 was dramatically restored by the introduction of the additional mutation of K25R (S33D+K25R), whereas the addition of the K36R mutation (S33D+K36R) did not increase the stability of S33D FOXL2 ( Fig. 4c ; lanes 4 versus 6 and 4 versus 8). This result implies a critical role of K25 in mediating the degradation of S33-hyperphosporylated FOXL2. In contrast, the enhanced stability of S33A FOXL2 was lost on the introduction of the K36R substitution (S33A+K36R), whereas the K25R mutation (S33A+K25R) did not alter S33A FOXL2 stability, suggesting a crucial role of K36 in maintaining the stability of S33-hypophosphorylated FOXL2 ( Fig. 4c ; lanes 10 versus 14 and 10 versus 12). The degrees of ubiquitination and SUMOylation of these FOXL2 mutants ( Fig. 4d ) correlated with their protein stability shown in Fig. 4c . These results indicate that K25 is a critical ubiquitin ligation site and that K36-mediated SUMOylation hampers FOXL2 ubiquitination. Thus, these data suggest that FOXL2 hyperphosphorylation at S33 decreases protein stability by stimulating FOXL2 ubiquitination, an effect that involves K25. Alternatively, the S33 underphosphorylation promotes FOXL2 stability by enhancing K36-mediated SUMOylation, hampering ubiquitin conjugation at K25. To determine how these PTMs affect FOXL2 activity, luciferase reporter and cell death assays were conducted by employing the mutants that were evaluated in Fig. 4d . The promoted luciferase activities of the S33A mutant on TNF-R1 , Fas , Caspase 8 , p21 and CYP19 were significantly attenuated by the introduction of the K36R mutation (S33A+K36R; Fig. 4e ). In contrast, the decreased luciferase activities of the S33D mutant were partially restored by the addition of the K25R mutation (S33D+K25R; Fig. 4e ). The effects of these mutations on cellular viability were in agreement with the observed modulation of the transcriptional activities, the S33A-induced increase in apoptosis was reduced by the additional mutation of K36R (S33A+K36R) and the S33D-induced decreased apoptotic activity was restored by the introduction of the K25R mutation ( Fig. 4f ). On the basis of these observations, a regulatory scheme of FOXL2 PTMs that regulate FOXL2 degradation was proposed: GSK3β-mediated S33 phosphorylation induces MDM2-mediated ubiquitin ligation at K25 and the phosphorylation opposes K36-involved SUMO conjugation; in contrast, UBC9-involved SUMO conjugation at K36 prevails when S33 is underphosphorylated, preventing FOXL2 ubiquitination ( Fig. 4g ). S33 hyperphosphorylation in patients with the C134W mutation Given that we observed diminished FOXL2 activities following GSK3β-mediated S33 phosphorylation, various FOXL2 mutants that are observed in GCT and blepharophimosis-ptosis-epicanthus inversus syndrome patients were ectopically expressed and evaluated for their differential S33 phosphorylation status. Among them, a specific and prominent increase in S33 phosphorylation was only observed in C134W FOXL2, which is present in GCT patients ( Fig. 5a ). An in vitro kinase assay clearly showed a stronger 32 P-incorporated band in C134W compared with WT FOXL2 ( Fig. 5b ). In addition, both in vitro and in vivo immunoprecipitations revealed that the C134W mutant exhibited a stronger direct interaction with GSK3β compared with the WT protein ( Fig. 5c,d ). Moreover, the interaction of C134W FOXL2 with MDM2 was significantly stronger compared with that of WT FOXL2 ( Fig. 5d ). As expected, C134W FOXL2 was more ubiquitinated and less SUMOylated than WT FOXL2 both in vivo and in vitro ( Fig. 5e,f ). These effects are likely to be S33 phosphorylation-dependent given that the introduction of the S33A mutation to C134W (C134W+S33A) abolished the differential ubiquitination and SUMOylation effects that were elicited by C134W ( Fig. 5e ). Similarly, the stability of the C134W mutant was also reduced ( Fig. 5g ), resulting in less efficient cell death activity ( Fig. 5h ). However, the introduction of the S33A substitution in the C134W mutant (C134W+S33A) completely restored cell death activity to the level of WT ( Fig. 5h ), implying that the defective cell death activity of C134W is primarily due to the phosphorylation of the S33 residue. In contrast, the FOXL2 mutant with alanine substituted at S263 (S263A), another phosphorylation site that was identified ( Supplementary Table S2 ), did not affect its ubiquitination ( Supplementary Fig. S3i ). 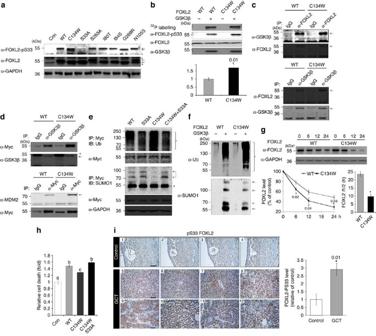Figure 5: Patients with C134W mutant-bearing GCTs exhibit hyperphosphorylated FOXL2 S33. (a) The levels of S33 phosphorylation on the ectopic expression of various FOXL2 mutants were compared by western blotting. (b) The hyperphosphorylation of S33 of C134W was confirmed using anin vitrokinase assay and immunoblot analyses. Equal amounts (2 μg) of purified WT and C134W proteins were incubated with active GSK3β protein (0.05 μg). A representative result is given. Quantitative analysis of S33-phosphorylated FOXL2 normalized to total FOXL2 levels (relative FOXL2-pS33 levels from three independent experiments is presented). (c)In vitrodirect interactions of recombinant GSK3β (0.05 μg) protein with 0.2 μg of purified WT or C134W FOXL2 proteins were compared by immunoprecipitation and western blot analyses. (d) Thein vivochanges in the binding capacity of C134W FOXL2 with GSK3β and MDM2 in comparison with WT FOXL2 were assessed using immunoprecipitation. Myc-tagged WT and C134W FOXL2 proteins were overexpressed in KGN cells. (e) The degrees of ubiquitination and SUMOylation of mutant FOXL2s were compared with WT FOXL2 by immunoprecipitation and western blot analyses. Mutant FOXL2 proteins were ectopically expressed in KGN cells, and the cells were incubated in the presence of MG132 (50 μM). (f) The increased ubiquitination and the decreased SUMOylation in the C134W mutant compared with WT were confirmedin vitro. Purified WT and C134W FOXL2 proteins (2 μg) were incubated with active GSK3β (0.05 μg) in the ubiquitination or SUMOylation reaction buffers. (g) The effect of C134W mutation on protein stability was assessed as described in the legend ofFig. 3a. Results (means±s.e.m.) are from three independent experiments. The statistically significant values are indicated with asterisks (P<0.05; Student’st-test). (h) The role of S33 phosphorylation in compromised cell death activity of C134W was determined using the C134W+S33A double mutant following transfection of KGN cells. Cell death was analysed according to the legend ofFig. 2b. (i) The immunohistochemical analysis of S33-phosphorylated FOXL2 in human GCTs (n=8) and controls (n=4) is shown. The GCTs analysed were all adult type possessing C134W. The staining intensities were quantified (means±s.e.m.) as described in the Methods section. The statistically significant values are indicated with asterisks (P<0.05; Student’st-test). Scale bar, 5 μm. Asterisk indicates nonspecific bands. Figure 5: Patients with C134W mutant-bearing GCTs exhibit hyperphosphorylated FOXL2 S33. ( a ) The levels of S33 phosphorylation on the ectopic expression of various FOXL2 mutants were compared by western blotting. ( b ) The hyperphosphorylation of S33 of C134W was confirmed using an in vitro kinase assay and immunoblot analyses. Equal amounts (2 μg) of purified WT and C134W proteins were incubated with active GSK3β protein (0.05 μg). A representative result is given. Quantitative analysis of S33-phosphorylated FOXL2 normalized to total FOXL2 levels (relative FOXL2-pS33 levels from three independent experiments is presented). ( c ) In vitro direct interactions of recombinant GSK3β (0.05 μg) protein with 0.2 μg of purified WT or C134W FOXL2 proteins were compared by immunoprecipitation and western blot analyses. ( d ) The in vivo changes in the binding capacity of C134W FOXL2 with GSK3β and MDM2 in comparison with WT FOXL2 were assessed using immunoprecipitation. Myc-tagged WT and C134W FOXL2 proteins were overexpressed in KGN cells. ( e ) The degrees of ubiquitination and SUMOylation of mutant FOXL2s were compared with WT FOXL2 by immunoprecipitation and western blot analyses. Mutant FOXL2 proteins were ectopically expressed in KGN cells, and the cells were incubated in the presence of MG132 (50 μM). ( f ) The increased ubiquitination and the decreased SUMOylation in the C134W mutant compared with WT were confirmed in vitro . Purified WT and C134W FOXL2 proteins (2 μg) were incubated with active GSK3β (0.05 μg) in the ubiquitination or SUMOylation reaction buffers. ( g ) The effect of C134W mutation on protein stability was assessed as described in the legend of Fig. 3a . Results (means±s.e.m.) are from three independent experiments. The statistically significant values are indicated with asterisks ( P <0.05; Student’s t -test). ( h ) The role of S33 phosphorylation in compromised cell death activity of C134W was determined using the C134W+S33A double mutant following transfection of KGN cells. Cell death was analysed according to the legend of Fig. 2b . ( i ) The immunohistochemical analysis of S33-phosphorylated FOXL2 in human GCTs ( n =8) and controls ( n =4) is shown. The GCTs analysed were all adult type possessing C134W. The staining intensities were quantified (means±s.e.m.) as described in the Methods section. The statistically significant values are indicated with asterisks ( P <0.05; Student’s t -test). Scale bar, 5 μm. Asterisk indicates nonspecific bands. Full size image Although the expression levels of endogenous FOXL2 were very low and not detected in KGN cells by western blot analysis ( Supplementary Fig. S4a ), we performed a series of experiments in both COV434 and rat primary granulosa cells to ensure that the experimental results obtained from KGN cells are not confounded by endogenously expressed FOXL2. Analogous results were obtained for GSK3β-dependent phosphorylation of FOXL2 and differential protein stability between WT and C134W FOXL2, as well as for the cell death activity of FOXL2 proteins on inhibition of GSK3β ( Supplementary Fig. S4b–g ). Of particular interest, the immunohistochemical analysis of human ovaries of patients with C134W-bearing GCTs and controls revealed that the ovaries of GCT patients exhibited significantly increased S33 phosphorylation by as much as threefold ( Fig. 5i ), whereas decreased FOXL2 expression in GCTs were observed ( Supplementary Fig. S5a ). The ratios of phospho-FOXL2 to FOXL2 in controls and GCTs assessed by immunohistochemical staining were 1.0±0.17 ( n =4) and 3.99±0.27 ( n =8), respectively ( Supplementary Fig. S5b ). To ensure the ovaries of follicular cysts that we used were appropriate as a control, we performed haematoxylin and eosin staining and immunohistochemistry of inhibin α on sections from the same tissues ( Supplementary Fig. S5c ). These results provide direct supporting evidence that S33 hyperphosphorylation of the C134W mutant probably contributes to GCT development. Enhanced tumorigenesis by C134W or S33D On the basis of these observations, we hypothesized that a molecular cue for the pathogenesis of C134W-bearing GCTs is the enhanced GSK3β-mediated S33 phosphorylation leading to reduced FOXL2 stability. To test this hypothesis, we established cell lines that stably overexpressed WT or mutant FOXL2 proteins. The results obtained using the stable cell lines were consistent with results from transiently transfected cells with respect to the status of S33 phosphorylation and FOXL2 expression level ( Fig. 6a ). Moreover, the augmented S33 phosphorylation of S33D and C134W mutants was effectively inhibited by the GSK3β inhibitor AR-A014418 ( Fig. 6a ). The effects on cell growth for these stable cells was also in agreement with data from transiently transfected cells, and the increased growth of cells that overexpressed either S33D or C134W was greatly inhibited by AR-A014418 ( Fig. 6b ). In contrast, the S33A stable cell line exhibited nearly no response to the same inhibitor ( Fig. 6b ). Differentially regulated expression of FOXL2 target genes in the established stable cells were confirmed by real-time PCR ( Supplementary Fig. S6 ). No significant difference was observed in both gel filtration analyses and circular dichroism profiles of the FH region of WT and C134W mutant ( Supplementary Fig. S7a,b ), and their homology models show that S33 is accommodated by the active cleft of GSK3β and W134 is exposed ( Supplementary Fig. S8a,b ). 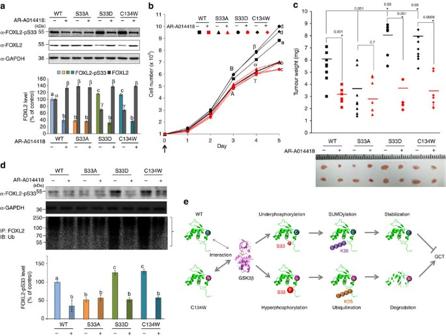Figure 6: C134W overexpression stimulates tumorigenesis and GSK3β inhibition suppresses tumour development. Stable cells that overexpress WT, S33A, S33D or C134W FOXL2 were produced. These cells were treated with 2 mg kg−1AR-A014418 or 0.1% dimethyl sulphoxide (DMSO) at the time of seeding the cells. (a) The changes in S33 phosphorylation and expression level of FOXL2 were determined by immunoblot analysis using anti-pS33 and anti-FOXL2 antibodies, respectively. Quantitative analysis of the S33-phosphorylated and the level of FOXL2 from three independent experiments is presented (lower panel). (b) The effects of S33 phosphorylation on cell death were measured. The results (means±s.e.m.) are from three independent experiments that were performed in triplicate. Statistically significant values at each time point are denoted with asterisks (P<0.05; Student–Newman–Keuls test). (c) The stable cells (2 × 107) that were generated were subcutaneously injected into mice twice over an interval of 2 weeks. Mice were injected with AR-A014418 (2 mg kg−1) or 0.1% DMSO every 24 h for 2 weeks, and the xenografts were excised and weighed. Each dot represents a tumour weight (n=8~9). Corresponding tumours that were excised from each group are shown in the lower panel. Statistical analysis was performed as described inb. Statistically significant values are indicated with asterisks (P<0.05; Student'st-test). (d) The changes in S33 phosphorylation of the excised tumours fromcwere determined using immunoblot analysis. Quantitative analysis of S33-phosphorylated FOXL2 level from three ovaries is presented (lower panel). Moreover, the changes in FOXL2 ubiquitination for the different mutants were assessed from pooled lysates that were prepared from four independent tumours fromcby immunoprecipitation and western blotting. Statistical analysis was performed as described inb. (e) A model of the mechanism by which the C134W mutation may lead to GCT development is proposed. Specifically, enhanced GSK3β-mediated S33 hyperphosphorylation is followed by MDM2-mediated proteasomal degradation, leading to GCT development. Figure 6: C134W overexpression stimulates tumorigenesis and GSK3β inhibition suppresses tumour development. Stable cells that overexpress WT, S33A, S33D or C134W FOXL2 were produced. These cells were treated with 2 mg kg −1 AR-A014418 or 0.1% dimethyl sulphoxide (DMSO) at the time of seeding the cells. ( a ) The changes in S33 phosphorylation and expression level of FOXL2 were determined by immunoblot analysis using anti-pS33 and anti-FOXL2 antibodies, respectively. Quantitative analysis of the S33-phosphorylated and the level of FOXL2 from three independent experiments is presented (lower panel). ( b ) The effects of S33 phosphorylation on cell death were measured. The results (means±s.e.m.) are from three independent experiments that were performed in triplicate. Statistically significant values at each time point are denoted with asterisks ( P <0.05; Student–Newman–Keuls test). ( c ) The stable cells (2 × 10 7 ) that were generated were subcutaneously injected into mice twice over an interval of 2 weeks. Mice were injected with AR-A014418 (2 mg kg −1 ) or 0.1% DMSO every 24 h for 2 weeks, and the xenografts were excised and weighed. Each dot represents a tumour weight ( n =8~9). Corresponding tumours that were excised from each group are shown in the lower panel. Statistical analysis was performed as described in b . Statistically significant values are indicated with asterisks ( P <0.05; Student's t -test). ( d ) The changes in S33 phosphorylation of the excised tumours from c were determined using immunoblot analysis. Quantitative analysis of S33-phosphorylated FOXL2 level from three ovaries is presented (lower panel). Moreover, the changes in FOXL2 ubiquitination for the different mutants were assessed from pooled lysates that were prepared from four independent tumours from c by immunoprecipitation and western blotting. Statistical analysis was performed as described in b . ( e ) A model of the mechanism by which the C134W mutation may lead to GCT development is proposed. Specifically, enhanced GSK3β-mediated S33 hyperphosphorylation is followed by MDM2-mediated proteasomal degradation, leading to GCT development. Full size image To further determine whether the altered cell death activities of the C134W and S33 mutants indeed affect GCT development in vivo , stably expressing KGN cells were injected into mice and their oncogenic activities were assessed. The xenograft of C134W-overexpressed KGN cells showed increased tumour weight compared with WT; a similar increase was observed for the S33D mutant ( Fig. 6c ). In striking contrast, xenograft formation was the least efficient with S33A mutant-overexpressing cells ( Fig. 6c ). In addition, injections of AR-A014418 significantly decreased the tumour weights from cells expressing C134W or S33D mutants but not the S33A mutant ( Fig. 6c ). Western blot analysis of tumours confirmed enhanced S33 phosphorylation following the injection of either C134W or S33D mutant-expressing cells, whereas negligible S33 phosphorylation was detected in tumours overexpressing the S33A mutant ( Fig. 6d ). Moreover, AR-A014418 injections resulted in significant attenuation of S33 phosphorylation, especially for C134W or S33D mutant-expressing cells ( Fig. 6d ). Strikingly, the amounts of ubiquitinated FOXL2 in tumours from each group correlated well with the degree of S33 phosphorylation ( Fig. 6d ). Although it has been clear that the FOXL2 C134W mutation is the major cause for GCT development [3] , [21] , [22] , [23] , [24] , [25] , [26] , [27] , the pathophysiological mechanism(s) responsible for FOXL2 C134W-mediated GCT are largely unknown. Here we identified distinctive PTMs of FOXL2 and the C134W mutant that involve differential GSK3β-mediated phosphorylation of S33. This residue serves as a phosphodegron, potentially accounting for the oncogenic property of the C134W mutant. Unlike many other targets of GSK3β, such as β-catenin [28] and Snail [28] , which require priming phosphorylation to allow GSK3β-mediated phosphorylation, GSK3β directly binds to the N-terminal region of FOXL2 without the requirement for priming. We also observed that the S33 phosphorylation of FOXL2 by GSK3β induces proteasomal degradation of FOXL2 in response to K25-linked ubiquitin conjugation. In contrast, the inhibition of S33 phosphorylation increased FOXL2 stability by promoting K36 SUMOylation, which hinders FOXL2 ubiquitination. These results indicate that the fate of FOXL2 is under the delicate control of sequential posttranslational regulatory events. Similarly, several proteins, including IκBα, HIF-1α, CREB, PCNA and Huntingtin, are also known to be regulated by conjugation to either ubiquitin or SUMO in an antagonistic manner [29] . Therefore, the mechanism of modulation of FOXL2 function by the hierarchic PTMs identified here may well provide a clue as to how this putative tumour suppressor is regulated. We also identified MDM2 as the E3 ligase of FOXL2 that is required for ubiquitin conjugation. MDM2-induced ubiquitination of other FH family transcription factors, including FOXO1, FOXO3A and FOXO4, has been previously demonstrated [30] , [31] . MDM2 physically associates with FOXL2; S33 phosphorylation allows for the stronger binding of MDM2 and subsequent FOXL2 polyubiquitination. In contrast, underphosphorylated FOXL2 at S33 preferentially binds to UBC9, an E2 ligase that is required for SUMO conjugation. This combined regulatory modification of FOXL2 is similar to the degradation of IκBα protein during the inflammatory response. In this context, phosphorylation by IκB kinase allows its β-TrCP-binding, ubiquitination and subsequent degradation, whereas IκBα SUMOylation promotes its stabilization [32] , [33] . The most significant result of this study is that the C134W mutation exhibits a different profile of PTMs compared with WT FOXL2, which could account for its tumorigenic properties. The C134W mutant interacts with GSK3β more strongly than the WT protein, resulting in FOXL2 hyperphosphorylation and enhanced association with MDM2, followed by a subsequent increase in ubiquitination and decrease in SUMOylation. Gel filtration analyses and circular dichroism profiles revealed no significant differences between the core domain (aa 43–144) of the two purified WT and C134W FOXL2 recombinant proteins ( Supplementary Fig. S7a,b ). Homology models of WT FOXL2 and the C134W mutant show that C134 is buried and the side chain of W134 is exposed to the solvent ( Supplementary Fig. S8a ). According to this docking model, the FOXL2 segment containing S33 is accommodated by the active site cleft of GSK3β and the FOXL2 FH domain is bound to a surface patch of GSK3β with FOXL2 W134 positioned at the binding interface ( Supplementary Fig. S8b ). The W134-mediated interaction between FOXL2 and GSK3β would facilitate the phosphorylation at S33 of FOXL2 by GSK3β. Although the precise underlying mechanism by which GSK3β binds more strongly to C134W than WT awaits further studies, based on our data we generated a model that may explain the mechanism by which the C134W mutation contributes to the development of GCT ( Fig. 6e ). Our findings regarding the degree of changes in PTMs and activities between WT and C134W FOXL2 are relatively modest. We think it is conceivable that a relatively moderate change in FOXL2 protein stability determines growth of GCT. This moderate but significant change in FOXL2 stability by the C134W mutation may explain the indolent nature of GCTs. GCT presentation in elderly women with median age of 50–54 years [2] may be the consequence of a longer duration required for granulosa cells to develop GCT owing to the slow accumulation of these moderate differences in the ovary. Other mutations in FOXL2 leading to more dramatic changes in transcriptional activity and induction of apoptosis than the C134W mutation were not found in GCT patients, indicating the detrimental effects of such mutations on normal ovarian development. This notion was supported by a recent report showing that FOXL2 ablation in granulosa cells in mice resulted in somatic sex reprogramming of adult ovaries to testes [13] . We think that relatively moderate changes in transcriptional activity and induction of apoptosis by decreased steady-state levels of FOXL2 in GCT patients are sufficient to maintain the persistent growth of GCT, whereas these levels of FOXL2 are required to carry out other essential functions such as folliculogenesis and the maintenance of female ovarian somatic cells. This study has implications for the field of cancer research as a whole by providing in vivo evidence, indicating that the status of S33 phosphorylation is proportional to the growth of GCT, and that GSK3β inhibition is an effective intervention for GCT therapy. At present, the applications of pharmacological inhibitors of GSK3β have been heavily focused on a small number of restricted disorders of the nervous system and type 2 diabetes [34] . This study suggests that GSK3β inhibitors can also be specific and effective tools for the inhibition of C134W-harbouring GCTs. Plasmid constructions The mutants pCMV-Myc-FOXL2 S33A, S33D, S263A, K25R, K36R, K48R, K54R, K87R and C134W+S33A construct were produced using a recombinant PCR technique using the following primers (Bioneer): FOXL2-F (5′-CTAGAATTCAAATGATGGCCAGCTACCCC-3′), S33A-F (5′-CCGGCCCCAGGCAAGGGCGGTGGGGGT-3′), S33D-F (5′-CCGCCGGATCCAGGCAAGGGCGGT-3′), FOXL2 S263A-F (5′-CAGGCCATGGCGCTGCCCCCCGGC-3′), S25R-F (5′-GGTCGCACAGTCAGAGAGCCAGAA-3′), S36R-F (5′-CCAGGCAGAGGCGGTGGGGGTGGC-3′), S48R-F (5′-GCCCCGGAGAGACCGGACCCG-3′), S54R-F (5′-CCGGACCCGGCGCAGAGACCC-3′), S87R-F (5′-ATCATCGCGAGATTCCCGTTC-3′), S87R-F (5′-ATCATCGCGAGATTCCCGTTC-3′), FOXL2 S33A-R (5′-ACCCCCACCGCCCTTGCCTGGGGCCGG-3′), FOXL2 S33D-R (5′-ACCGCCCTTGCCTGGATCCGGCGG-3′), FOXL2 263A-R (5′-GCCGGGGGGCAGCGCCATGGCCTG-3′), FOXL2-K25R-R (5′-TTCTGGCTCTCTGACTGTGCGACC-3′), FOXL2-K36R-R (5′-GCCACCCCCACCGCCTCTGCCTGG-3′), FOXL2-K48R-R (5′-CGGGTCCGGTCTCTCCGGGGC-3′), FOXL2-K54R-R (5′-GGGTCTCTGCGCCGGGTCCGG-3′), FOXL2-K87R-R (5′-GAACGGGAATCTCGCGATGAT-3′) and FOXL2-R (5′-CTACTCGAGTCAGAGATCGAGGCGCGAATG-3′). The pCMV-HA-SUMO1 expression construct was produced using the primers SUMO1-F (5′-CTAGAATTCAAATGTCCGAGGAGAAGCCCAA-3′) with SUMO1-R (5′-CTACTCGAGCTAGAAACTGTGCCC-3′) and the pCMV-HA Ubiquitin expression construct was made using the primers Ubiquitin-F (5′-CTAGAATTCAAATGCAGATTTTCGT-3′) with Ubiquitin-R (5′-CTACTCGAGTTACTTGTCTTCTGG-3′). The PCR products were digested with Eco RI and Xho I (Enzynomics), and ligated into the pCMV-Myc, HA (Clontech). The pcDNA3 MDM2 expression constructs were generated using the following primers: MDM2-F (5′-CTAGAATTCATGGTGAGGAGCAGGC-3′), MDM2-R (5′- CTACTCGAGCTAGGGGAAATAAGTTAGC-3′), MDM2 Δ209–274-F (5′-CTCTGTGTGTATCAGATGA-3′) and MDM2 Δ209–274-R (5′-TCATCTGATACACACGAGA-3′). The PCR products were digested with Eco RI and Xho I (Enzynomics) and ligated into the pcDNA3 (Clontech). Various E3 ligase-coding plasmids were generous gifts from Dr In Kyoung Lim (Ajou University; Flag-SKP2), Dr Kang Yell Choi (Yonsei University; Flag-β-TrCP) and Dr Suk-Chul Bae (Chungbuk University; Flag-ARFBP1). RNA interference The siRNA target sequence of GSK3β was 5′-AAGAGACGAUGGACUUCCGAU-3′. The control siRNAs used were 5′-CCUACGCCACCAAUUUCGU-3′ and 5′-ACGAAAUUGGUGGCGUAGG-3′. MDM2 siRNA was purchased (Bioneer). The sense and antisense oligonucleotides were annealed in the presence of Annealing Buffer (Bioneer). Generation of the anti-phospho-S33 antibody The polyclonal phospho-S33 FOXL2 antibody was raised and purified against a synthetic human FOXL2 peptide (GRTVKEPEGPPPS(p)PGKGGGGGGGTAPEKPDPAQKPPYSYV; AbFrontier) and the antibody titre was determined using a peptide-specific enzyme-linked immunosorbent assay. Cell culture and transfection Human adult-type GCT-derived KGN cells bearing the C134W mutation were cultured and transfected by electroporation as described previously [8] . Human COV434 cells derived from juvenile GCT and 293T cells were cultured in DMEM media and transfected by Lipofectamine 2000 (Invitrogen). The isolation, culture and transfection of rat primary granulosa cells were performed as we previously reported [35] . In brief, 21-day-old rats were injected subcutaneously with 20 mg of diethylstilbesterol (Sigma) daily for 3 days. Ovaries were isolated, placed in a Petri dish containing Leibovitz medium (Gibco BRL) and 0.1% BSA (Bovogen), transferred to a new dish and punctured with a 1-ml syringe needle (Kovax). Granulosa cells were collected by centrifugation (160 g ) for 3 min and washed with McCoy medium (Welgene). The primary granulosa cells (1 × 10 6 ) were transfected with 3 μg of plasmid DNA using Metafectene (Biontex) following the manufacturer’s instructions. The animals were treated according to the experimental protocol approved by the Chung-Ang University Institutional Animal Care and Use Committee. Subcellular fractionation The 293T or KGN cells (1 × 10 8 ) were transfected with 30 μg of plasmids that encoded FOXL2 WT or C134W. After 24 h of incubation, the cells were washed twice with cold PBS and treated with cytosolic extraction buffer A for 5 min at room temperature (10 mM HEPES, pH 7.9, 10 mM KCl and 0.1 mM EDTA). This buffer contained 1 mM dithiothreitol (DTT), 10% IGEPAL CA-630 and a protease inhibitor cocktail. After centrifugation at 1,000 g for 5 min at 4 °C, the supernatants were removed and the pellets that contained the nuclear factions were solubilized in nuclear lysis buffer B (20 mM HEPES, pH 7.9, 0.4 M NaCl, 1 mM EDTA and 10% glycerol) that contained 1 mM DTT and a protease inhibitor cocktail. The nuclear proteins were then obtained from centrifugation at 10,000 g for 10 min at 4 °C. Mass spectrometry analysis The nuclear proteins from the subcellular fractionation of 293T cells overexpressing either WT or C134W FOXL2 were enriched via immunoprecipitation with anti-FOXL2 antibody (AbFrontier). The proteins were alkylated with 100 mM iodoacetamide in the dark after treatment with 10 mM DTT at 60 °C for 15 min and cooling at room temperature. The proteins were then precipitated with 2 M trichloroacetic acid and washed twice with cold 80% acetone. The air-dried proteins were digested overnight with 1:20 sequencing grade trypsin (Promega) at 37 °C. The tryptic peptides were acidified with 0.2% trifluoroacetic acid to clean them using Vivapure C18 microspin columns (Vivascience) and dried in vacuo . Dried peptides were dissolved in 10 μl 0.4% acetic acid and were analysed using a Thermo Scientific LTQ-Velos mass spectrometer that was connected to a reversed-phase Magic C18AQ column (ID75 × OD150 μm × L75 mm) and an EASY-nLC 1000 system that operated at a flow rate of 0.3 μl min −1 . The chromatographic condition was a 90-min linear gradient from 5 to 40% acetonitrile in a 0.1% formic acid buffer solution. This step was followed by a 10-min column wash with an 80% acetonitrile concentration and a 20-min re-equilibration to the initial buffer condition. Survey full-scan mass spectrometry spectra ( m/z 300–2,000) were performed to determine the MS2 precursor ions and charge states. The MS2 spectra of the five most intense ions from the preview survey scan were acquired in the ion trap with the following options: isolation width, ±1.5 m/z ; collision energy, 35%; and dynamic exclusion duration, 30 s. The acquired mass spectral data were manipulated with Xcalibur version 2.1 software and identified from a non-redundant sequence database of Homo sapiens (women) using X! Tandem at http://ppp.thegpm.org/ . The following options were used: precursor mass tolerance, 4 Da; fragment mass error, 0.4 Da; fixed carbamidomethylation (C); refinements of partial cleavage sites and potential modifications for (di)oxidation (M, W), phosphorylation (S, T, Y) or ubiquitination (diglycyl-K); and peptide and protein log(e)-values of <−2. Western blot analysis and immunoprecipitation Cell lysates were prepared 24 h following transfection, subjected to electrophoresis and immunoblotted with the respective antibodies. The membranes were then stripped and sequentially reprobed with other antibodies. The inputs were one-tenth the amount of the immunoprecipitates. The purchased antibodies included anti-Myc (Clontech, 1:500), anti-FOXL2 (Abcam, 1:500), anti-GSK3β (Cell Signaling, 1:1,000), anti-phospho-GSK3β (Cell Signaling, 1:1,000), anti-Flag (Sigma, 1:1,000), anti-SUMO1 (Santa Cruz Biotechnology, 1:1,000), anti-Ubiquitin (Santa Cruz Biotechnology, 1:1,000), anti-MDM2 (Santa Cruz Biotechnology, 1:1,000), anti-β actin (Santa Cruz Biotechnology, 1:3,000), anti-H2B (Santa Cruz Biotechnology, 1:1,000), anti-inhibin α (Santa Cruz Biotechnology, 1:100) and anti-GAPDH (AbFrontier, 1:3,000). The immunoprecipitation analyses were conducted according to a previous report [35] . The protein bands in the gel were detected with a Bio-Rad ChemiDoc system (Bio-Rad Laboratories) and the intensity of each band was quantitated with OptiQuant. The production of recombinant FOXL2 proteins His-tagged full-length FOXL2 proteins were produced as we described previously [35] . To construct the vector expressing the core domain (aa 43–144) of FOXL2 (WT and C134W), the corresponding DNA region was amplified using pET28a-FOXL2 or pET28a-FOXL2 C134W plasmids as a template and then inserted into Eco RI and Xho I sites of the pPROEX-HTA vector (Invitrogen). To express the proteins, the Escherichia coli BL21(DE3) cells harbouring the vectors were cultured in Luria broth medium that contained 50 μg ml −1 ampicillin at 37 °C until OD 600 =0.6. After induction with 0.5 mM isopropyl-β- D -thiogalactoside, the cells were further grown at 30 °C for 5 h and collected by centrifugation. The cell pellet was resuspended with 20 mM Tris (pH 8.0) buffer that contained 150 mM NaCl and 2 mM 2-mercaptoethanol, and then disrupted with sonication. The cell debris was removed by centrifugation and applied to Ni-NTA agarose on an Econo-Pac column (Bio-Rad Laboratories). After washing with 20 mM Tris buffer containing 250 mM NaCl, 20 mM imidazole and 2 mM 2-mercaptoethanol, the proteins were eluted with 20 mM Tris buffer that contained 250 mM NaCl, 200 mM imidazole and 2 mM 2-mercaptoethanol. To remove the imidazole, the eluted fractions were dialysed against 20 mM Tris buffer (pH 8.0) that contained 250 mM NaCl and 2 mM 2-mercaptoethanol. The proteins were concentrated to 2 mg ml −1 by size-exclusion chromatography using Centricon YM-50 filter devices (Millipore). Luciferase assay Luciferase assays were conducted using the reporter constructs with the TNF-R1 , Fas , Caspase 8 , p21 or CYP19 promoters, as previously described [8] , [35] . KGN cells (4 × 10 5 ) were transfected with 170 ng of pCMV β-galactosidase plasmid (Clontech), 300 ng of TNF-R1 , Fas , Caspase 8 or p21 -responsive luciferase reporters, and plasmids coding FOXL2 WT or mutants using a Neon system (Invitrogen), followed by incubation on 12-well plates containing fresh DMEM/F12 medium for 24 h. Promoter activities were measured using Luciferase assay system kit (Promega). The absorbance was measured with the FlexStation3 microplate reader (Molecular Devices). The results are given as the relative luciferase activity in fold change following normalization to β-gal expression. RT–PCR and real-time PCR analyses The reverse transcription of extracted total RNA and subsequent real-time PCR were conducted as previously reported [8] . Quantification of transcripts was normalized to glyceraldehydes 3-phosphate dehydrogenase (GAPDH). Nucleotide sequences of the primers used were as follows: GAPDH (5′-AGCCAAAAGGGTCATCATCTCT-3′ and 5′-AGGGGCCATCCACAGTCTT-3′), TNF-R1 (5′-CCAAATGGGGGAGTGAGAGG-3′ and 5′-AAAGGCAAAGACCAAAGAAAATGA-3′), FAS (5′-TGAAGGACATGGCTTAGAAGTG-3′ and 5′-GGTGCAAGGGTCACAGTGTT-3′), Caspase 8 (5′-AGCCCCACGATGACTGCACA-3′ and 5′-GGGCCTCCTGTCCATCAGTGC-3′), p21 (5′-TGTCCGTCAGAACCCATGC-3′ and 5′-AAAGTCGAAGTTCCATCGCTC-3′) and CYP19 (5′-TGCCACCATGCCAGTCCTGC-3′ and 5′-TGCCGTGGGAGATGAGGGGT-3′). In vitro kinase assay The purified recombinant FOXL2 proteins were incubated with an active GSK3β recombinant protein (Sigma) in the presence of 50 μM ATP or 5 μCi[γ- 32 P]ATP (Sigma) in a kinase buffer for 30 min at 30 °C. The kinase reaction was initiated by the addition of an equal volume of 10 × reaction buffer (100 mM HEPES, pH 7.4, 100 mM MgCl 2 and 10 mM DTT). 32 P-labelled FOXL2 protein was visualized by autoradiography (AgenBio) and immunoblotting was performed with the appropriate antibodies of anti-pS33-FOXL2 (1:500), anti-FOXL2 (Abcam; 1:500) and anti-GSK3β (Cell Signaling; 1:1,000). Cell viability assay Cell viability was measured using the CellTiter-Glo assay kit (Promega) 24 h following the transfection of the KGN cells, according to the manufacturer’s instructions. Cell death was analysed and presented as fold change compared with the control condition. Stoichiometry of GSK3β-mediated FOXL2 phosphorylation In vitro kinase assay of FOXL2 (1 μg) by GSK3β (0.2 μg) was performed in 10 × reaction buffer (100 mM HEPES, pH 7.4, 100 mM MgCl 2 , 10 mM DTT and 0.001647 μM [γ- 32 P]ATP) at different time points. Aliquots were applied to electrophoresis. The gel was stained with Coomassie blue, dried and subjected to autoradiography. Chromatin immunoprecipitation and quantitative RT–PCR Chromatin immunoprecipitation experiments were conducted as we reported previously [35] . The precipitated DNA fragments were amplified using specific primers for TNF-R1 , Fas , Caspase 8 and p21 that encompass the putative FOXL2-binding sequences (−751 to −532 of TNF-R1 , −452 to −263 of Fas , −666 to −382 of Caspase 8 and −805 to −554 of p21 ) via real-time PCRs, and the data were analysed as provided by the manufacturer (Qiagen). Nucleotide sequences of the primers used were as follows: TNF-R1 (5′-AGGGGAGGATTACTAAGGGA-3′ and 5′-TCCAATTCAGAATGCTTAGC-3′), FAS (5′-CCTCACCTGAAGTGAGCATG-3′ and 5′-AGGATGGGAAGGAAGCCTCG-3′), Caspase 8 (5′-AAGGTCACGCAGCTAGTA AGT-3′ and 5′-GTGAAAACTTCTCCCATGGCCT-3′) and p21 (5′- CTGCAACCACAGGGATTTCT-3′ and 5′-AGAAGCACCTGGAGCACCTA-3′). Ubiquitination assay In vivo ubiquitination was determined by immunoprecipitation and western blot analyses using KGN cells that were cultured in the presence of 50 μM of MG132. For the in vitro ubiquitination assay, the auto-ubiquitinylation kit (BML-UW0970, Enzo Life Sciences) and recombinant E1-3 ligases (UBA5, UbcH5c and MDM2; Abcam) were used as suggested by the manufacturer. SUMOylation assay The in vivo SUMOylation analysis was conducted according to the methods described in a previous report [14] . The in vitro SUMOylation assay was performed using a SUMOylation kit (BML-UW8955, Enzo Life Sciences) as described previously [16] . Human GCT sampling and immunohistochemistry The cases were collected at the Bundang CHA General Hospital, CHA University, from 2005 to 2010. The protocols and consent forms were approved by the Bundang CHA general Hospital Institutional Review Board, and all cases were reviewed by a pathologist. The expression patterns of S33-phosphorylated FOXL2 and FOXL2 in eight GCTs and control ovaries that were obtained from patients who underwent salpingo-oophorectomy due to follicular cysts were analysed by immunohistology, as reported previously [23] . Paraffin-embedded tissues were sectioned to a thickness of 5 μm using a FINESSEE microtome (Thermo Scientific) and deparaffinized. The sections were rehydrated, immersed in an antigen-retrieval solution (0.01 M sodium citrate and 0.05% Tween 20, pH 6.0) and microwaved for 10 min (100 °C at 600 W). Endogenous peroxidase was blocked by immersing the sections in a 3% hydrogen peroxidase solution (Duksan) for 10 min, followed by rinsing in PBS. Nonspecific staining was blocked with 2.5% normal horse serum (Vector Laboratories) for 1 h at room temperature. The sections were then incubated with polyclonal a rabbit polyclonal pS33-FOXL2 antibody (1:100) in the antibody diluent (Dako) for 24 h at 4 °C. For the incubation with secondary antibody, the LSAB+ System-HRP (Dako) was used as directed by the manufacturer. All sections were counterstained with Mayer’s haematoxylin solution for 5 min. The slides were then dehydrated and mounted for microscopic observation. Control ovaries have homozygote for 402C, whereas all of the GCTs used were heterozygote of 402C and 402G. Quantification of the immunohistochemistry data was conducted as previously reported [36] . In brief, the images were acquired at X200 using Olympus CKX41 microscope (Olympus) connected to Sony power shot G12 digital camera (Sony) and saved as joint photographic experts group format in size of 4–5 MB. After the image acquisition, percentage of labelled cells and intensity of immunostaining were obtained using Matlab 2013a (MathWorks). The unit of quantified data generated from Matlab is mathematical energy, E M (energy unit/pixel). Haematoxylin and eosin staining was conducted as previously described [37] . Basic clinical data for human samples are presented in Supplementary Table S3 . In vivo xenograft mouse model KGN cells (4 × 10 7 ) were subcutaneously injected into female BALB/c nu/nu immunodeficient 5-week-old mice (Central Lab Animal Inc.) with a weight range of 18–20 g. After 4 weeks, the GSK3β inhibitor AR-A014418 (2 mg kg −1 ) was intraperitoneally injected ten times into the KGN cell-injected site over 2 weeks. The animal protocol was approved by the Chung-Ang University Institutional Animal Care and Use Committee, and the animals were treated as described in the protocol. Statistical analysis Multiple comparison analyses of values were performed with the Student–Newman–Keuls test (SAS), and significance of values was analysed by comparison with controls with Student’s t -test. The data represent the means±s.e.m. and P <0.05 was considered to be statistically significant. The P -values of significant results are shown. How to cite this article: Kim, J.-H. et al . FOXL2 posttranslational modifications mediated by GSK3β determine the growth of granulosa cell tumours. Nat. Commun. 5:2936 doi: 10.1038/ncomms3936 (2014).